Phylogenetic applications of whole Y-chromosome sequences and the Near Eastern origin of Ashkenazi Levites Previous Y-chromosome studies have demonstrated that Ashkenazi Levites, members of a paternally inherited Jewish priestly caste, display a distinctive founder event within R1a, the most prevalent Y-chromosome haplogroup in Eastern Europe. Here we report the analysis of 16 whole R1 sequences and show that a set of 19 unique nucleotide substitutions defines the Ashkenazi R1a lineage. While our survey of one of these, M582, in 2,834 R1a samples reveals its absence in 922 Eastern Europeans, we show it is present in all sampled R1a Ashkenazi Levites, as well as in 33.8% of other R1a Ashkenazi Jewish males and 5.9% of 303 R1a Near Eastern males, where it shows considerably higher diversity. Moreover, the M582 lineage also occurs at low frequencies in non-Ashkenazi Jewish populations. In contrast to the previously suggested Eastern European origin for Ashkenazi Levites, the current data are indicative of a geographic source of the Levite founder lineage in the Near East and its likely presence among pre-Diaspora Hebrews. Whole Y-chromosome sequencing holds the promise of stretching the human paternal phylogeny to its maximal resolution. The absence of recombination enables all Y-chromosome sequences to be placed within a single phylogenetic tree. Clearly, a single locus hierarchy may oversimplify the demographic history of a particular individual. However, in contrast to the autosomes, the ordering of the accumulated sequence variants since the most recent common ancestor is preserved. Due to this molecular encapsulation of human male demographic history, the human Y-chromosome phylogeny has become one of the pillars of archaeogenetics and is particularly informative for testing hypotheses based on genealogical information [1] , [2] . While some Y-chromosome haplogroups show pronounced affiliation to a single continent [3] , [4] , [5] , [6] , many others, particularly those within the broadly defined Old World (Eurasia), have a wide cross-continental range of distribution [7] , [8] . Accordingly, paternal population genetic heritage cannot rely solely on the presence of a given list of haplogroups within the populations of interest, but must consider the haplogroup frequencies comprising the respective paternal gene pools [9] , [10] . At the individual or paternal pedigree level, this means that haplogroups shared between populations do not confirm an unequivocal paternal ancestry to a particular population within the haplogroup’s geographic range of distribution. To distinguish between two populations, an informative marker is one that approaches fixation in one group and is absent in another [11] . Such markers should be forthcoming from whole-genome sequences, to be followed by genotyping in larger panels to more precisely delineate patterns of restricted geographic and/or population specificity. Here, we describe the identification of such a Y-chromosome marker from whole Y-chromosome sequencing, which, despite its overall low frequency across Eurasia, coincides with a restricted set of populations within the Near East and among Jews. The widespread Eurasian distribution zone of haplogroup R1a has been mapped for over a decade [8] , [10] , [12] , [13] since the first reports that the M17 deletion grouped Y-chromosomes into a monophyletic clade that exceeded 30% frequency in some Asian populations [14] and over 50% in Eastern Europe [15] . Several single nucleotide polymorphisms (SNPs) phylogenetically equivalent to M17, such as M198, are now known [16] . Nonetheless, the internal structure of the R1a haplogroup has long resisted fractionation until the recent separation of its post-glacial European and Asian coancestry was partially achieved with the discovery of the M458 SNP [16] . Efforts to clarify the genetic ancestry of East European Jews have been ongoing [17] . Progress towards disentangling the internal structure of haplogroup R1a is integral to our ability to resolve the debate over the geographic origin of the Ashkenazi Jewish Levite founding lineage, which is defined by a short tandem repeat (STR)-based haplotype that is rare elsewhere [18] . The Jewish people can be categorized in a number of ways. For example, one arrangement is into Ashkenazi [19] and non-Ashkenazi [20] , which separates Jews recently descended from Central and Eastern Europe from other Jewish Diaspora communities. In addition, Jewish heritage recognizes three paternally inherited castes, Cohen, Levite and Israelite, of which the first two are considered priesthood lineages [18] , [21] , [22] , [23] . Levites comprise ~4% of the male Jewish population and display genetic evidence for multiple recent origins, with Ashkenazi Levites reported to carry a particularly high frequency (>50%) of a distinctive STR-based lineage nested within haplogroup R1a-M198 (refs 18 , 24 , 25 ). Previous studies have demonstrated that haplogroup R1a is rare in other Jewish castes, other Jewish communities and in non-Jewish groups of Near Eastern origin [18] , [21] . However, it is found at high frequency in populations of eastern European origin [16] , [18] , [26] , [27] . The greatly elevated frequency of haplogroup R1a-M198 within Ashkenazi Levites, their compact network of STR haplotypes and the recent coalescence time, suggest a founder event specific to the Ashkenazi Levites and a paternal ancestor shared by more than half of contemporary Ashkenazi Levites. The long residence of Ashkenazi Jews in Eastern Europe and the high frequency of haplogroup R1a in the same region suggested that the founder might be of non-Jewish European ancestry, whose descendants were able to assume Levite status. However, because of the paucity of distinctive internal substructure of haplogroup R1a, it was not possible to suggest a particular European source population nor to test the hypothesis of a Turkic-speaking Khazar ancestor, which has been proposed in light of the narrative that members of the Khazar ruling class may have converted to Judaism in the 8th or 9th century [18] . Here we study the phylogenetic origin of the Ashkenazi Levite lineage at the whole Y-chromosome level. First, to allow the appropriate phylogenetic context and depth, we reconstruct the phylogeny of the parental haplogroup R1 using a total of nine R1a and seven R1b whole Y-chromosome sequences. Next, we launch a phylogenetically informative large-scale population-based study in order to resolve the geographic origin of the Ashkenazi Levite founding lineage within the transcontinental distribution range of haplogroup R1a. We find that the set of nucleotide substitutions that characterizes 91.9% of Ashkenazi R1a lineages occurs at low frequencies in non-Ashkenazi Jewish and Near Eastern populations while being absent in Eastern Europe host populations, which were previously considered to be the most likely source for the majority of Ashkenazi Levite Y-chromosome lineages. Haplogroup R1 whole Y-chromosome phylogeny We have determined at high coverage the sequence of eight Jewish and five non-Jewish Y-chromosomes ( Supplementary Table S1 ) belonging to haplogroup R1 ( Fig. 1a and Supplementary Fig. S1 ). We reconstructed the phylogenetic relationships of the newly sequenced samples in the context of three other available high coverage sequences from this haplogroup using binary SNP data ( Supplementary Data 1 ) from a total of 8.97 Mbp of sequence from the non-recombining region of nine Y-chromosomes [28] . For both sub-clades of R1, most Jewish sequences cluster separately from the clades that in previous studies have been shown to be common in Europe: in R1b where more than 90% of European lineages are within the L11/L52 clade [29] , three of the newly sequenced Jewish Y-chromosomes cluster within its copanion clade defined by the Z2105 mutation; in R1a where the majority of European individuals belong to the S198 (ref. 30 ) and M458 branches [16] , all four newly sequenced Jewish Y-chromosomes fall into the clade defined by Z94 mutation. Furthermore, two Ashkenazi R1a chromosomes were found to share 19 SNPs ( Supplementary Fig. S1 ) of which six were found to be shared with an Iberian individual from the 1,000 Genomes database. One of the mutations defining this clade including Ashkenazi and Iberian samples, which we designate M582 (AKA CTS2253), was subjected to genotyping in 2,834 R1a samples to determine its geographic distribution, diversity and divergence times. 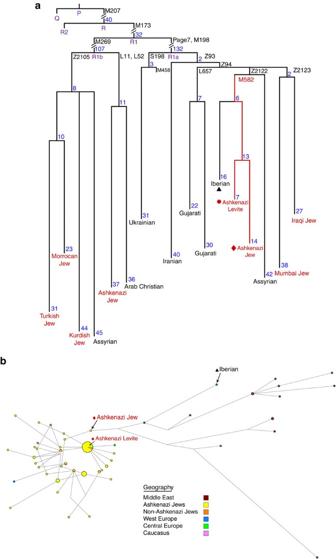Figure 1: Y-chromosome haplogroup R1 phylogeny and haplogroup R1a-M582 STR haplotypes diversity. (a) Schematic representation of haplogroup R1 phylogeny as reconstructed from 16 whole Y-chromosome sequences. The detailed figure is shown inSupplementary Fig. S1. (b) MJN of haplogroup R1a-M582 samples using the 19 Y-chromosome STRs: DYS19, DYS388, DYS389I, DYS389II, DYS390, DYS391, DYS392, DYS393, DYS439, DYS461=A7.2, DYS385a, DYS385b, DYS437, DYS438, DYS448, DYS456, DYS458, DYS635 and Y GATA H4. Circles represent haplotypes, with area proportional to frequency and coloured according to population, as shown in the legend. The smallest circles represent singletons. The branch lengths are proportional to the number of STRs separating the nodes. The allocations of the Iberian (HG01617), Ashkenazi Levite (16207) and Ashkenazi Jewish (P3) whole-genome samples are marked in both panels of the figure by the triangle, flower and diamond signs, respectively. Figure 1: Y-chromosome haplogroup R1 phylogeny and haplogroup R1a-M582 STR haplotypes diversity. ( a ) Schematic representation of haplogroup R1 phylogeny as reconstructed from 16 whole Y-chromosome sequences. The detailed figure is shown in Supplementary Fig. S1 . ( b ) MJN of haplogroup R1a-M582 samples using the 19 Y-chromosome STRs: DYS19, DYS388, DYS389I, DYS389II, DYS390, DYS391, DYS392, DYS393, DYS439, DYS461=A7.2, DYS385a, DYS385b, DYS437, DYS438, DYS448, DYS456, DYS458, DYS635 and Y GATA H4. Circles represent haplotypes, with area proportional to frequency and coloured according to population, as shown in the legend. The smallest circles represent singletons. The branch lengths are proportional to the number of STRs separating the nodes. The allocations of the Iberian (HG01617), Ashkenazi Levite (16207) and Ashkenazi Jewish (P3) whole-genome samples are marked in both panels of the figure by the triangle, flower and diamond signs, respectively. Full size image Population-based survey for R1a-M582 Among non-Jewish populations, the overall frequency of R1a-M582 was found to be 0.15% (22/15,138) and among R1a-M198 it was 0.81% (22/2,711) ( Table 1 ). The geographic distribution of the haplogroup appears to be limited to West Eurasia, as we did not observe it in South Asia, Central Asia or Southern Siberia. Haplogroup R1a-M582 was only sporadically observed in Europe, the Diaspora residence of Ashkenazi Jews. Notably, it was not identified among 2,149 samples (including 922 R1a-M198) of non-Jews from East Europe, where the Ashkenazi Jewish community flourished in recent centuries ( Table 1 ). While the frequency of R1a in the paternal gene pool of Eastern European Slavonic and non-Slavonic peoples [16] , [18] , [31] reaches as high or higher than 50%, the deeper phylogenetic resolution reported here renders the presumption that similarly high frequencies of R1a among Ashkenazi Levites reflect substantial gene flow or a founder effect from their hosts highly unlikely. Within 1,068 West/North European samples (106 R1a-M198), M582 was observed in just one German sample, and among 3,756 Central/South European samples (710 R1a-M198), it was found only in one Hungarian and one Slovakian sample ( Table 1 ). It is important to note that many of the samples from individuals of European descent from Germany, The Netherlands, England, Ireland and Norway were collected in USA without ethnicity or religious affiliation information, so some of them might represent contemporary Ashkenazi Jews residing in the United States. As such, our results are likely more conservative because fewer of our R1a-M582 samples actually have non-Jewish European ancestry. Among 3,739 Near Eastern samples (303 R1a-M198), R1a-M582 was identified in various populations, with the highest frequency occurring within Iranians collected from the southeastern Kerman population who self-identified as Persians, northwestern Iranian Azeri and in Cilician Anatolian Kurds, at 2.86%, 2.50% and 2.83%, respectively ( Table 1 ). In contrast, among 2,164 samples from the Caucasus (211 R1a-M198), R1a-M582 was found in just one Nogay sample ( Table 1 ). As the overall frequencies obtained for R1a-M582 were low, we applied Fisher's exact test to verify that the different sample sizes did not bias our results ( Supplementary Table S2 ). Out of a total of eight tests for the entire population, all but one was significant at the nominal 0.05 level, and all but three were still significant after a Bonferroni correction. For the R1a-M198 samples only, all eight tests were significant at the 0.05 level and all but one significant after Bonferroni correction. Table 1 R1a clade frequencies in different regions and populations. Full size table Among Jews ( Table 1 ), the overall frequency of R1a-M582 was 6.33% (90/1,421), while representing 73.17% (90/123) of the R1a-M198 chromosomes. Two factors must be considered when interpreting these frequencies: the known founder effect previously reported for Ashkenazi Levites [18] and the differing degrees of demographic information available for our 1,421 Jewish samples, compiled from various sampling campaigns [18] , [21] , [24] . For part of the sample, only the name of the community and not the paternal caste was documented. Hence, some Ashkenazi samples carrying haplogroup R1a-M582 might be undocumented Levites. Other collections specifically recruited Cohanim and Levites, so their inclusion in this study is likely to increase our overall estimate of R1a-M582 frequency among Ashkenazi Jews. These biases should affect the non-Ashkenazi Jewish data set, comprising 821 samples, to a lesser degree. Of the 821 non-Ashkenazi Jewish samples, 36 (4.38%) belonged to haplogroup R1a, and ten (1.22%) belonged to R1a-M582 ( Table 2 ). These frequencies are similar to R1a-M582 frequencies observed in non-Jewish Near Eastern populations. Of the 10 non-Ashkenazi R1a-M582 individuals, two were from the North African Algerian Jewish community, six belonged to Spanish expulsion descendent communities of Slovenia, Turkey and Bulgaria, and two were from individuals reporting their last known parental origin as Israel. Significantly, all eight individuals for whom caste information was available self-identified as Levites. Caste information was unavailable for the two Bulgarian individuals ( Supplementary Data 2 ). Moreover, out of nine R1a-M198 non-Ashkenazi Levites, eight were R1a-M582. Among the 600 Ashkenazi Jews, 87 belonged to haplogroup R1a-M198, and of these, 80 (91.95%) were confirmed to belong to haplogroup R1a-M582 ( Table 2 ). The Ashkenazi samples included a total of 279 Israelites, 110 Cohens, 97 Levites and 114 unclassified samples in which the counts and frequencies of haplogroup R1a-M198/R1a-M582 were 12 (4.3%)/7 (2.5%), 1 (0.9%)/1 (0.9%), 63 (64.9%)/63 (64.9%) and 11 (9.6%)/9 (7.9%), respectively ( Table 2 ). Remarkably, all Ashkenazi Levite R1a samples belonged to haplogroup R1a-M582, and this haplogroup is virtually absent among members of the Cohen caste. Table 2 R1a clade frequencies within Jewish castes. Full size table STR-based network analysis Patterns of Y-chromosome STR diversity are useful for identifying additional population substructure among individuals belonging to the same haplogroup [32] . Of the 90 Jewish R1a-M582 samples reported herein, STR haplotypes were obtained for 86 of them ( Supplementary Data 2 ). The Median Joining Network (MJN) demonstrated one clear cluster and a more differentiated set of chromosomes within haplogroup R1a-M582 ( Fig. 1b ). The first cluster, referred to below as the Ashkenazi cluster, includes Ashkenazi Levites, Ashkenazi non-Levites, non-Ashkenazi Jews and Europeans. This Ashkenazi cluster demonstrates a star-like pattern with Ashkenazi Levites, non-Ashkenazi Jews and Central European samples sharing the modal haplotype. The more differentiated set of chromosomes, referred to below as the Near Eastern set, include populations sampled from an area covering contemporary Iran and eastern Anatolia (Turkey), including southeastern Iranian Kerman, northwestern Iranian Azeri, Kurds from the historic Cilician part of Anatolia and Kazakhstan, one Nogay, and a single Ashkenazi Jew—the index case (P3, Supplementary Table S1 ). This Near Eastern set demonstrates a non-star-like pattern with multiple mutational events separating the various component haplotypes. These results strongly suggest and are consistent with a split in the R1a-M582 haplogroup, which has not yet been identified. Furthermore, DYS456 had significant discriminatory power within haplogroup R1a-M582 for separating the Ashkenazi Levite cluster from the Near Eastern set of haplotypes ( Fig. 1b ). Only one STR profile, obtained from the Ashkenazi Jewish R1a-M582 whole-genome sample, exhibited 15 repeats rather than 14 repeats at locus DYS456, and this haplotype was two mutational steps removed from the Levite modal haplotype. While the allocations of the Ashkenazi Levite, Ashkenazi Jewish and Iberian whole-genome samples are marked on the MJN ( Fig. 1b ), the latter two samples were not part of our population set, and accordingly they were excluded from our population-based analyses. Dating the Ashkenazi Levite lineage Assuming a mutation rate of 1 × 10 −9 per base pair per year in the 8.97 Mbp region [28] of the X-chromosome degenerate non-recombining regions of the Y-chromosome, we estimated the divergence time of the two Ashkenazi M582 whole sequences that differed at 21 positions as 1,200 (SE 300) years. This divergence time represents a lower bound for the age of R1a-M582 because the time estimate was based on just two individual sequences that may share a more recent common ancestor than the rest of the Levites. The Iberian M582 lineage was excluded from age calculations because its low coverage made calling private mutations uncertain. The upper bound for the age of the M582 clade was estimated as the divergence time of the two Ashkenazi M582 lineages and the Assyrian R1a-Z2122(xM582) sequence, yielding an estimate of 4,000 (SE 300) years. Relying on larger sample sizes, we also estimated the coalescence time of the R1a-M582 lineages from STR data. The coalescence age of the Near Eastern cluster was 11.3±4.1 kya, as compared with a coalescence time of 2.4±1.0 kya for the Ashkenazi Jewish cluster. The coalescence age calculated from Ashkenazi Levites alone was 2.6±1.2 kya, which was similar to the age of 3.1±1.5 kya obtained for non-Ashkenazi Jews. Estimates of the coalescent times must be viewed with caution, in part because of uncertainties involving an appropriate choice of Y-chromosome STR mutation rate, but comparisons between groups are informative [33] . Furthermore, the much lower variance among Jews relative to that observed for the Near Eastern cluster is striking. Our coalescence analysis should be interpreted cautiously in light of some pertinent caveats. First, our whole Y-chromosome-based analysis relied on results from next generation sequencing. Several factors indicate high sequencing accuracy was achieved, such as the high coverage of the obtained positions, the ability to reconstruct the haplogroup R1 phylogeny, the identification of known SNPs of phylogenetic relevancy, the fact that the studied genetic locus is uniploid, and the ability to obtain the same positions from different samples using different platforms. However, Sanger-type sequencing was not used to validate all of the positions used to reconstruct our phylogeny. Therefore, both false-positive and false-negative calls might render our estimates provisional. Second, it is also possible that results obtained from using the different genotyping platforms of Complete Genomics and Illumina might have introduced biases into our variant calls. Third, our STR-based coalescence analysis used an evolutionary mutation rate as one of its priors, although considerable controversy exists regarding whether a pedigree-based mutation rate is more appropriate. We opted to use the evolutionary rate because the samples used in the analysis represented very different ancestries and were therefore unlikely to share genealogical ties in recent generations. Last, coalescence analysis is prone to additional biasing factors still much debated in the literature, such as the correct mutation rate and the actual generation time. Our data necessitate revising the current hypotheses regarding the origins of the Ashkenazi Levite founding lineage. Consistent with the previous conclusions [18] , the tight cluster of Ashkenazi Levite R1a-M582 haplotypes strongly indicates a recent origin from a single common ancestor who, according to our provisional dating, lived ~1.5–2.5 kya. Importantly, this young STR-based age estimate is now further supported by evidence from Y-chromosome sequences. However, the previously proposed Eastern European origin of this lineage is no longer tenable given that our data suggest haplogroup R1a-M582 actually originated in the Near East [18] . The higher R1a-M582 diversities and frequencies observed among Near Eastern populations indicate R1a-M582 originated in this geographic region. While this conclusion is independent of our findings from Jews, the mere existence of the haplogroup among Jews actually lends further support. However, as the frequencies of R1a-M582 were low overall, we first assessed and demonstrated that the frequencies observed in the different continental/sub-continental regions ( Table 1 ) were statistically significant considering the different sample sizes ( Supplementary Table S2 ), which we now discuss in detail. Considering the historical records of Ashkenazi Jews, three potential geographic sources should be considered: the Near East, which was the geographic location for the ancient Hebrews; Europe, which was the residence of the Ashkenazi Jewish Diaspora and the region in which they evolved for nearly two millennia; and the region overlapping with the no longer extant mid-11th Century Khazarian Khaganate, whose ruling class has been suggested to have converted to Judaism [18] . Our data render the latter source highly unlikely since the Khazarian Khaganate overlapped with the Northern Pontic-Caspian steppe and the North Caucasus region, in which just one Nogay sample carried the R1a-M582 haplogroup ( Table 1 ). Furthermore, the Nogays, formerly a powerful Kipchak Turkic-speaking nomadic confederation, are relatively recent inhabitants of the Caucasus, and the STR haplotype of the sole R1a-M582 Nogay sample lies outside of the Levite cluster. Had the Caucasus region been the source for the Ashkenazi modal lineage, we likely would have found R1a-M582 Y-chromosomes in some of its 20 local populations examined in our sample of more than 2,000 Y-chromosomes ( Table 1 ). As previously suggested, the European and particularly, the Eastern European paternal gene pool was seen as a natural and highly plausible source for the Ashkenazi Levite lineage as both the Ashkenazi community and haplogroup R1a frequencies peak in this region. But surprisingly, haplogroup R1a-M582 was not detected in non-Jewish Eastern European samples and was found only in singleton samples in various Central and Western European populations ( Table 1 ). The direction of gene flow involving the Ashkenazi Levite R1a-M582 lineage warrants discussion. The presence of haplogroup R1a-M582 at minute frequencies among Europeans could theoretically suggest introgression into the Ashkenazi Levite community and subsequent expansion among Ashkenazi Levites. Alternatively, the European samples can represent Ashkenazi admixture into the general European gene pool due to assimilation that has occurred in Western Europe throughout the centuries. While it is impossible to refute the former, a few arguments render the latter more likely. The European samples carrying haplogroup R1a-M582 haplotypes add no further diversity to that found among Ashkenazi Jews, despite having been identified at different European locations. These haplotypes are actually identical or one step removed from the Levite modal haplotype. If haplogroup R1a-M582 were of general ancient European ancestry, we would have observed at least some baseline diversity and genetic distance expressed in a few STR-based mutational events between the lineages evolving in the general European gene pool and the one lineage whose evolution is confined to the Ashkenazi samples. While this pattern could not be demonstrated among Europeans, it was clearly evident among Near Eastern samples. Near Eastern populations are the only populations in which haplogroup R1a-M582 was found at significant frequencies ( Table 1 ). Moreover, the representative samples displayed substantial diversity even within this geographic region ( Fig. 1b ). Higher frequencies and diversities often suggest lineage autochthony. Hence, we can assess whether or not the origin of haplogroup R1a-M582 is in present-day Iran and eastern Anatolia, or rather the broader region of the Near East. Our data demonstrate the occurrence of R1a-M582 among different Iranian populations, among Kurds from Cilician Anatolia and Kazakhstan, and among Ashkenazi and non-Ashkenazi Jews. These observations, and the STR network delineating an internal R1a-M582 structure, might attest to a broad Near Eastern distribution range of this minor haplogroup that survived to the present day at low frequencies among Iranian Kerman, Iranian Azeri, Kurds and Jews. Haplogroup R1a-M582 was not detected in samples from Iraq or among Bedouins, Druze and Palestinians sampled in Israel. Additional samples from the region between the Levant and Iraq, such as from Syria, were not available. The identification of an R1a-M582 chromosome in the Iberian sample from the 1,000 Genome Project might represent the legacy of Jews or Moors in Iberia [34] . The STR pattern obtained for this sample is more compatible with the latter ( Fig. 1b ). The MJN also demonstrates that the STR profile obtained for the whole Ashkenazi Jewish sample is within the range of variation observed in the Near Eastern set of chromosomes ( Fig. 1b ). While this finding can merely represent a mutational event within a set of fast evolving STRs, it can also suggest the existence of multiple R1a-M582 sub-clades within the presumed ancestral Levantine deme of contemporary Ashkenazi Jews. Notably, the only non-M582 sample we identified within the Z2122 haplogroup ( Fig. 1a and Supplementary Fig. S1 ) corresponds to an individual from the Aramaic speaking population claiming descent from the contemporary ancient Assyrians. Aramaic and Hebrew, the two ancient Western Semitic languages that are still spoken are thought to have diverged ~3,500–4,000 years ago [35] , in a time frame coinciding with time estimate suggested above for the age of R1a-Z2122 haplogroup. Taken together, this line of evidence supports a Near Eastern origin for haplogroup R1a-M582, and hence the Ashkenazi Levite lineage as well. Another notable observation regards the distribution of haplogroup R1a-M582 among Ashkenazi and non-Ashkenazi Levites. While R1a-M582 occurs at 64.9% (63/97) among Ashkenazi Levites, it comprises just 15.7% (8/51) of the non-Ashkenazi Levite paternal gene pool ( Table 2 ). Among non-Ashkenazi Jews, R1a-M582 was observed only in Levites, and the observed sub-haplogroup shares the same STR signature as that seen in Ashkenazi Levites. A few demographic scenarios can account for this observation. Clearly, a joint Levantine origin before the Diaspora split into the Ashkenazi and non-Ashkenazi Jews must be considered. Under this scenario, this particular R1a-M582 Levite lineage existed among the ancient Hebrews and was carried to the various Jewish Diaspora communities in a manner similar to that of the Cohen Modal Haplotype [21] , [22] , [23] . However, recent studies of genome-wide diversity point to recent shared Levant ancestries and a close genetic proximity among members of Ashkenazi, North African and Spanish Exile Jewish communities [17] , [36] , [37] . Similarly, some of the mitochondrial DNA Ashkenazi founding lineages are also found among Spanish Exiles [20] . Therefore, another possible scenario is that of continuous gene flow between Ashkenazi, North African and Spanish Exile Jewish communities. Under this scenario, Ashkenazi Levites must have repeatedly and episodically introgressed into non-Ashkenazi communities, maintaining their Levite status while abandoning their Ashkenazi affiliation. The haplogroup distribution pattern observed for the Ashkenazi Levite lineage does not seem to be restricted to haplogroup R1a chromosomes. While haplogroup R1a is the most prevalent in East Europe, it is its companion haplogroup, R1b, that is the most frequent among West Europeans [38] . Similar to haplogroup R1a, haplogroup R1b frequencies are also found at low frequencies among non-Europeans, including Jews [39] . Based on distinct STR patterns, it has been suggested that some of the Jewish R1b chromosomes may have a West European origin and that some might be of Near Eastern origin [34] . Our sequence data are compatible with this suggestion as the Kurdish, Moroccan and Turkish Jewish R1b lineages for which whole Y-chromosome data was determined to coincide with a different branch than the one which is common in Europe ( Fig. 1a ). Intriguingly, we also noticed that like the R1a subclade, the particular subclade within R1b is also shared by Jews and a Y-chromosome, sampled in Aramaic speaking Assyrian descendants. In contrast, one Ashkenazi Jewish and one Arab Christian R1b lineages seem to be nested with the European R1b-L52 haplogroup. Estimating the proportion of haplogroup R1b chromosomes among Jews and in particular among Ashkenazi Jews of Levantine origin remains the scope of further studies. In summary, we have circumscribed the geography of marker M582 within the broad distribution zone of R1a-M198* lineages. We have shown it to be a minor haplogroup that is primarily shared among Iranian Kerman, Iranian Azeri, Kurds, Ashkenazi Jews and non-Ashkenazi Jews, and that it is virtually absent in the Caucasus region, Europe, South Asia, and southern Siberia. Thus, in contrast to previous suggestions regarding the origin of this Ashkenazi Levite founding lineage, we conclude that haplogroup R1a-M582 was likely carried into Europe by Jewish migrants and that it expanded among Ashkenazi Levites during their subsequent Diaspora period in a region that is incidentally dominated by other R1a parahaplogroups that coalesce with R1a-M582 prior to the establishment of the Jewish people. The existence of the R1a-M582 lineage within non-Ashkenazi Levites from different Jewish communities suggests it to either be a pre-Diaspora Hebrew Levite lineage or that continuous gene flow existed between Jewish communities, presumably, from Ashkenazi to non-Ashkenazi Jews. Our case study of Ashkenazi Levites is a vivid example of the ability to refine haplogroup structure and trace subtle signals of gene flow when sufficiently resolved data are available at the genomic and population levels. Preliminary screening of haplogroup R1a markers Whole-genome sequencing, privately obtained by an individual of Ashkenazi Jewish (Israelite) ancestry ( Fig. 1 , Supplementary Fig. S1 ), created the opportunity to address the topic of Ashkenazi Levite paternal heritage. Following Stanford University Human Subjects Internal Revenue Board approval, the list of all Y-chromosome SNP assignments was extracted from the whole-genome data and a saliva sample for DNA extraction was donated for validation and further analysis. This individual’s assignment to haplogroup R1a-M198*(xM458, M434) was confirmed using standard PCR-based genotyping assays [16] . The list contained SNPs previously undocumented on the genetic genealogy aggregator ISOGG web site. These putatively private alleles were then intersected with publically available low coverage Y-chromosome sequence data from the 1,000 Genomes Project ( http://www.1000genomes.org/data ). One of the Ashkenazi Jewish Y-chromosome SNPs appeared to be shared with a single sample from the Iberian population in Spain and hence labelled as potentially non-private. Accordingly, we initially screened a set of haplogroup R1a-M198 samples from the HGDP CEPH panel (Russia, Orkney Island, Caucasus, Israel and five ethnic groups from Pakistan), which was further augmented with Turks, Iranians and Greeks [16] . Since this marker was ascertained in the genome of an individual of Ashkenazi Jewish ancestry carrying an R1a Y-chromosome [18] , we also genotyped it in a small set of 13 Ashkenazi Levite known to belong to the same haplogroup [18] . As M582 was detected in all 13 Ashkenazi Levites and in one Iranian Kerman sample, a phylogenetic study of the Ashkenazi Levite lineage at the whole Y-chromosome level and a large-scale genotyping on all samples available to us followed. Whole Y-chromosome sequencing and phylogeny reconstruction Supplementary Table S1 details the information for each of the sixteen samples included in this study of which thirteen are first reported herein. Supplementary Data 1 outlines the reference and the alternative alleles for all markers discovered in the sequencing campaign. To reconstruct the phylogeny of haplogroup R1a-M198, we evaluated the two Gujarati R1a individuals sequenced by Complete Genomics [40] and the single Iberian individual sample reported as part of the 1,000 genome project using the Illumina platform [41] . Next, we identified all haplogroup R1a-M198 in all population sample collections available to us and chose seven additional samples for whole-genome sequencing. Samples were chosen to include a wide range of haplogroup R1a-M198 internal variation on the basis of previously available STR haplotypes ( Supplementary Data 2 ), populations and geographic regions relevant to the question of the origin on the Ashkenazi Levite lineage. Accordingly, within Ashkenazi Jews, one sample was from an Ashkenazi Levite carrying the Levite modal haplotype as inferred from STR analysis and one was the Israelite Ashkenazi Jew available from our preliminary work. One Iraqi Jew and one Mumbai Jew were included to allow a general understanding of the R1a-M198 variation within the Jewish world. Similarly, one Assyrian, one Iranian and one Ukrainian samples were chosen to grossly represent the large regions that might be relevant to the understating of the Ashkenazi Levite origin including the Near East and East Europe. In addition, and to accurately confirm our ability to reliably reconstruct the root of haplogroup R1a-M198 within its ancestral R1a, we studied a total of six haplogroup R1b-M269 samples from Near Eastern populations for which the current available public data is scant. It is also worth noting that the quality and source of DNA available to us had a significant role in our ability to include samples in our whole-genome sequencing campaign. In some cases, when samples of sufficient quality were unavailable from our population collections, new blood samples were collected from individuals self-affiliating with these populations to identify individuals carrying R1a-M198 individuals. Accordingly, Supplementary Table S1 details which samples are from our population data set and which are from other non-random collections. All samples reported herein were derived from blood samples that were collected with informed consent according to procedures approved by the Institutional Human Subjects Review Committees in their respective locations. All sixteen samples were used to reconstruct haplogroup R1 phylogeny ( Supplementary Fig. S1 ). The whole-genome sequences of the eight Jewish and five non-Jewish male individuals belonging to Y-chromosome haplogroup R1 were determined at high coverage using genomic DNA extracted from blood. High-quality variants mapping to Y-chromosome were extracted for downstream analyses. All but one sample were sequenced at Complete Genomics with Y-chromosome coverage >20 × and one Ashkenazi Jewish R1a-M582 sample was sequenced with Illumina HiSeq 2000 at 14 × coverage. Alignment and allele calling were performed using Complete Genomics pipelines and CGAtools. The Illumina sequence genomic library was prepared using the Epicentre Nextera Sample Preparation Kit. Paired-end reads were sequenced using four Illumina HiSeq 2000 lanes. Aligned coverage for the Y-chromosome was 14 × (ref. 42 ). Raw variant calls were generated using Broad Institute's GATK v4 best practices pipeline [43] , [44] , including read deduplication, base quality recalibration and local realignment around indels. In phylogenetic analyses we also used publicly available data from two Gujarati R1a individuals sequenced by Complete Genomics [40] . We filtered the data to exclude regions of poor mapping efficiency due to structural variation and focused on the nine X-chromosome degenerate non-recombining regions [28] that altogether encompass 8.97 Mbp of the Y-chromosome sequence. We also excluded from the analyses insertions, deletions and multistate SNPs. The one additional sample from an Iberian individual available from the 1,000 genome project is shown in our phylogeny ( Supplementary Fig. S1 ) but not included in our coalescence analysis because of its low coverage. We generated maximum-parsimony, neighbor-joining and minimum evolution trees in MEGA [45] for the high coverage Y-chromosome sequences. All trees generated were identical in topology. The consensus tree was rooted with haplogroup Q sequence from the Complete Genomics public data ( http://www.completegenomics.com/public-data/ ). The Build 37 coordinates of non-recurrent mutations defining branches within haplogroups R1a and R1b are shown in Supplementary Fig. S1 . Population collection and genotyping We investigated a total of 15,138 non-Jewish individuals from Europe, the Near East, the Caucasus and Asia available to us. This sample set included 2,711 individuals belonging to haplogroup R1a [16] , [27] , [46] , [47] , [48] , [49] , [50] , [51] , [52] . A total of 1,421 Jewish samples from across the entire range of Diaspora Jewish communities were included [18] , [21] , [24] , [39] . All samples were hierarchically screened for the haplogroup R1a defining markers M198 or M17 (ref. 16 ) and then to M582, which represents one of the 19 binary SNPs comprising the root of haplogroup R1a-M582 in which the Ashkenazi Levite lineage is nested. M582 is a g.14,236,070T>G transversion according to GRCh37/hg19 assembly version. M582 was genotyped by RFLP assay using Tsp509I enzyme following amplification with primers 5′-3′: F: 5′-GAGGCTGCAGTGAGCTATGAC-3′ and R: 5′-GTCACCTGCTTGGTAAAGATGAC-3′. Table 1 summarizes the populations used and the frequencies of haplogroup R1a-M198 and its descendant sub-haplogroup R1a-M582 within each population. To evaluate the significance of differences in prevalence of the R1a-M582 allele between Near Eastern populations and the other non-Jewish populations in our data, we utilized Fisher's exact test for comparisons of prevalence of R1a-M582 within the entire population sample and also within R1a-M198 samples only ( Supplementary Table S2 ). To assess the genetic distance between the Ashkenazi Levite R1a-M582 haplotypes and all other Jewish or non-Jewish M582 haplotypes from all geographic regions, we used a set of 19 Y-chromosome STRs ( Supplementary Data 2 ). This set of 19 Y-chromosome STRs could not be fully resolved in ten of the Jewish and five on the non-Jewish R1a-M582 samples due to DNA quantity and quality limitations. Previously reported datasets [16] , [18] were merged to obtain uniform STR haplotype profiles comprising the following 19 markers: DYS19, DYS388, DYS389I, DYS389II, DYS390, DYS391, DYS392, DYS393, DYS439, DYS461=A7.2, DYS385a, DYS385b, DYS437, DYS438, DYS448, DYS456, DYS458, DYS635, and Y GATA H4. In addition, the same 19 Y-chromosome STRs were assessed in the Ashkenazi Jewish and the Iberian samples (Coriell #HGO1617) which are not part of our population collection ( Supplementary Data 2 ). Age estimates using STRs and whole Y-chromosome variation MJN was generated using the recommended default settings of Network 4.6.1.1 but allowing a higher weight to DYS456, which proved to be particularly informative in our data set. Next, coalescent times (Td) [53] , [54] of haplogroup R1a-M582 and its sub-clusters were estimated using an evolutionary effective mutation rate of 6.9 × 10 −4 per 25 year generation for the following original set of 10 Y-chromosome STRs: DYS19, DYS388, DYS389I, DYS389II, DYS390, DYS391, DYS392, DYS393, DYS439, DYS461 (TAGA counts). For estimating the divergence times of the whole Y-chromosome sequences using the rho statistic [55] , [56] , we assumed mutation rate of 1 × 10 −9 per base pair per year [57] . STR profiles obtained from our whole-genome samples that are not part of our population set were not included in the calculations. Accession codes : The whole Y-chromosomes sequences have been deposited to the European Nucleotide Archive under accession code PRJEB4991 . How to cite this article : Rootsi, S. et al. Phylogenetic applications of whole Y-chromosome sequences and the Near Eastern origin of Ashkenazi Levites. Nat. Commun. 4:2928 doi: 10.1038/ncomms3928 (2013).